MicroRNA-378 controls classical brown fat expansion to counteract obesity Both classical brown adipocytes and brown-like beige adipocytes are considered as promising therapeutic targets for obesity; however, their development, relative importance and functional coordination are not well understood. Here we show that a modest expression of miR-378/378* in adipose tissue specifically increases classical brown fat (BAT) mass, but not white fat (WAT) mass. Remarkably, BAT expansion, rather than miR-378 per se , suppresses formation of beige adipocytes in subcutaneous WAT. Despite this negative feedback, the expanded BAT depot is sufficient to prevent both genetic and high-fat diet-induced obesity. At the molecular level, we find that miR-378 targets phosphodiesterase Pde1b in BAT but not in WAT. Indeed, miR-378 and Pde1b inversely regulate brown adipogenesis in vitro in the absence of phosphodiesterase inhibitor isobutylmethylxanthine. Our work identifies miR-378 as a key regulatory component underlying classical BAT-specific expansion and obesity resistance, and adds novel insights into the physiological crosstalk between BAT and WAT. Classical brown fat (BAT), primary located in the interscapular region of many mammals, has long been well recognized as an organ specialized for heat production, a property that is attributed to its extensive vascularization and sympathetic innervation, high mitochondrial density and oxidative capacity, and abundant expression of uncoupling protein-1 ( Ucp1 ) [1] . In addition, certain white fat (WAT) depots, such as subcutaneous inguinal WAT (iWAT), possess a subpopulation of adipocytes called beige or brite cells that confer plasticity and can be induced to brown-like adipocytes in response to various stimuli [2] , [3] , [4] , [5] , [6] . Both classical BAT and beige adipocytes are found in adult humans and their mass and/or activity are inversely correlated with body mass index [6] , [7] , [8] , [9] , [10] , [11] , [12] , [13] , [14] , [15] , [16] . These findings lead to the proposal that increasing BAT mass and/or activity or converting WAT adipocytes to beige adipocytes might be a promising therapeutic strategy for obesity and metabolic diseases, an idea that has gained strong support from numerous studies performed in rodents [17] , [18] , [19] . However, in many of these studies, a concomitant increase of activities of both classical BAT and beige adipocytes has been observed; hence, their relative contributions to obesity resistance are not fully understood [17] , [18] , [20] , and it remains to be determined whether and to what extent of expansion of classical BAT alone is sufficient to prevent obesity. Moreover, how the functions of classical BAT and beige adipocytes are coordinated are largely unclear. Adipogenesis of both WAT and BAT is driven by a Ppar γ transcriptional cascade, and many signalling molecules impinge upon the Ppar γ pathway to modulate adipogenesis [21] , [22] , [23] , [24] . Among them is cAMP second messenger. cAMP is turned over by members in the cyclic nucleotide phosphodiesterase (Pde) superfamily [25] , and for this reason, a nonselective PDE enzyme inhibitor isobutylmethylxanthine (IBMX) has been widely used to promote fat cell differentiation in vitro . However, how the activities of Pde enzymes are naturally attenuated during adipocyte differentiation is unknown. Brown and white adipogenesis are also specified by separate genetic entities. For example, a few genes have been shown to selectively operate in brown adipocytes to promote their adipogenesis [26] , [27] , [28] , [29] , [30] , [31] , [32] . For some of these genes such as C/EBP β, Ebf2 and Orexin , the lack of adipogenic effects on white adipocytes is due to either their low expression levels or absence of intact signalling transduction pathways, which ultimately fail to activate Ppar γ. On the other hand, co-factor Tle3 facilitates white adipogenesis by competing with Prdm16 for its interaction with PPAR γ [33] . Clearly, identifying additional regulatory components governing fat type-specific development and understanding their mechanisms of action are of great biomedical importance. MicroRNAs (miRNAs) are endogenous, noncoding small RNAs that control multiple developmental and cellular processes. miRNAs posttranscriptionally regulate gene expression through complementary base pairing between its seed sequence and 3′ untranslated region (UTR) of target mRNAs, triggering mRNA destabilization or translational repression [34] , [35] . miRNA targets are highly tissue- or cell type-dependent and one miRNA can have different functions by targeting different mRNAs in different tissues [34] , [36] , [37] . Several groups have investigated the importance of BAT-selectively expressed miRNAs in brown adipogenesis. These studies reveal that miR-155 and miR-133a/b inhibit brown adipogenesis [38] , [39] , [40] , [41] , and miR-193b-365 cluster enhances both brown and white adipogenesis [42] , suggesting diverse roles of miRNAs in BAT development. Despite these progresses, to date, miRNAs that positively control BAT-specific development have not been identified. Here we report that a modest expression of miR-378, at least in part, by targeting Pde Pde1b promotes BAT-specific expansion, which offers complete resistance to both genetic and high-fat diet-induced obesity. Surprisingly, BAT expansion, but not miR-378 per se , leads to suppression of development of beige adipocytes. Our work reveals a fat type-specific action of miR-378 in control of adipose development and obesity resistance, and provides insights into the physiological crosstalk between BAT and WAT. miR-378 transgene in adipose tissue expands classical BAT To begin investigating potential functions of miRNAs in BAT, we measured the expression of a total of 688 miRNAs in BAT and gonadal WAT by quantitative PCR with reverse transcription (RT–qPCR; Fig. 1a and Supplementary Data 1 ). miRNAs that displayed significantly higher level in BAT were selected and further examined for their expression in other tissues. Although, as noted previously [43] , most of our selected miRNAs are in fact skeletal muscle-specific miRNAs, three miRNAs, miR-378, miR-193b and miR-1941-3p, were highly enriched in BAT ( Fig. 1b ) [42] . Interestingly, none of these three miRNAs was induced by acute cold exposure ( Fig. 1c ). miR-378 was of particular interest, as it is induced during brown adipogenesis ( Fig. 1d,e ) and resides in the sense strand of the first intron of Pgc-1β, which is a transcriptional co-activator that regulates mitochondrial biogenesis and brown fat-specific gene expression [44] . In addition to miR-378, miR-378*, produced from the passenger strand of the 22 nucleotide RNA duplex, was detected in BAT at a very low level. 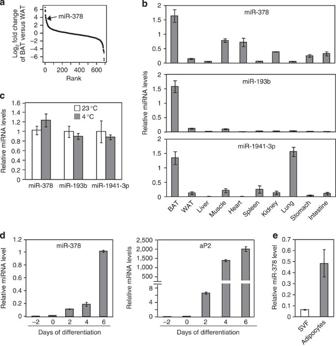Figure 1: Screening for BAT-selective miRNAs. (a) miRNAs were ranked in order of differential expression between BAT and gonadal WAT (n=5 mice, 10-week-old male mice). (b) miRNA tissue expression profile analysed by quantitative RT–PCR;n=5 mice (10-week-old male mice). (c) miRNA levels in BAT at 23 °C and at 4 °C (6 h);n=5 mice per group (10-week-old male mice). (d) miR-378 (left) andaP2mRNA (right) levels during brown fat cells differentiation. (e) miR-378 level in stromal vascular fraction (SVF) and mature adipocytes isolated from BAT of wild-type mice. All data are mean±s.e. Figure 1: Screening for BAT-selective miRNAs. ( a ) miRNAs were ranked in order of differential expression between BAT and gonadal WAT ( n =5 mice, 10-week-old male mice). ( b ) miRNA tissue expression profile analysed by quantitative RT–PCR; n =5 mice (10-week-old male mice). ( c ) miRNA levels in BAT at 23 °C and at 4 °C (6 h); n =5 mice per group (10-week-old male mice). ( d ) miR-378 (left) and aP2 mRNA (right) levels during brown fat cells differentiation. ( e ) miR-378 level in stromal vascular fraction (SVF) and mature adipocytes isolated from BAT of wild-type mice. All data are mean±s.e. Full size image To pinpoint the physiological role of miR-378, we generated transgenic mice ectopically expressing the miR-378 locus under the control of the aP2 promoter [45] ( Fig. 2a ), given that endogenous aP2 and miR-378 displayed a similar expression pattern during brown adipogenesis ( Fig. 1d ). The levels of miR-378 in the transgenic mice were about 3.3-fold in BAT and 3- to 10-fold in WAT, compared with the control littermates ( Fig. 2b ). Similar folds of miR-378* expression were observed ( Supplementary Fig. 1 ), thus total level of miR-378* remained extremely low. On a normal chow diet, the transgenic mice did not show any noticeable difference in outward appearance. Their body weights as well as food intakes were similar ( Fig. 2c,d ). However, upon dissection, it was evident that BAT was enlarged ( Fig. 2e ). We observed a 44% increase of BAT mass in female and a 35% increase in male transgenic mice ( Fig. 2f ). Surprisingly, both inguinal and gonadal WAT depots were significantly reduced ( Fig. 2e,f ). Other organs such as liver, skeletal muscle and heart showed no weight difference ( Fig. 2g ), and levels of circulating triglycerides, free fatty acids and glucose were normal ( Fig. 2h ). We also obtained a second miR-378 transgenic line, which displayed a similar BAT expansion phenotype and other phenotypes examined, albeit to a less extent, presumably due to a lower transgene expression ( Fig. 2i ). We thus characterized the first transgenic line in detail. In addition, we have generated aP2 promoter-driven miR-1941-3p transgenic mice and no BAT expansion phenotype was found. Together, we conclude that a very modest ectopic expression of miR-378 locus in adipose tissue results in a BAT-specific expansion accompanied with diminished WAT depots. 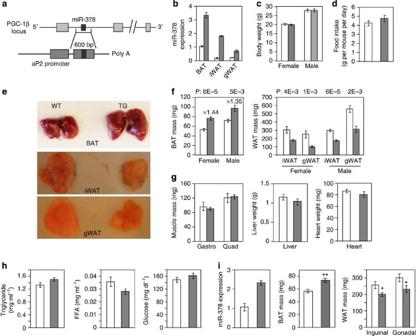Figure 2: Modest transgenic expression of miR-378 in adipose tissue produces a BAT-specific expansion. Empty bar, wild-type mice (WT); Grey bar, transgenic mice (TG). Mice were fed a normal chow diet. (a) Outline of miR-378/378* transgenic construct. (b) qPCR analysis of miR-378 levels in 9-week-old male WT and TG mice (n=3 mice per group). iWAT, subcutaneous inguinal WAT; gWAT, gonadal WAT. (c) Body weights. Female,n=10–12 mice per group (9-week-old mice); male,n=6 mice per group (14-week-old mice). (d) Food intake.n=5 male mice per group (10-week-old mice). (e,f) BAT and WAT mass. Female,n=10–12 mice per group (9-week-old mice); male,n=6 mice per group (14-week-old mice).Pvalues (TG versus WT, two-tailed Student’st-test) are indicated on top of the panels. (g) Liver, skeletal muscle and heart weights from mice ind. Gastro, gastrocnemius muscle; quad, quadriceps muscle. (h) Circulating triglycerides, free fatty acids and glucose levels.n=6–8 mice per group (14-week-old male mice). (i) miR-378 expression and BAT expansion in a second miR-378 transgenic line.n=6 mice per group (9-week-old male mice). *P<0.05, **P<0.005 (two-tailed Student’st-test). All data are mean±s.e. Figure 2: Modest transgenic expression of miR-378 in adipose tissue produces a BAT-specific expansion. Empty bar, wild-type mice (WT); Grey bar, transgenic mice (TG). Mice were fed a normal chow diet. ( a ) Outline of miR-378/378* transgenic construct. ( b ) qPCR analysis of miR-378 levels in 9-week-old male WT and TG mice ( n =3 mice per group). iWAT, subcutaneous inguinal WAT; gWAT, gonadal WAT. ( c ) Body weights. Female, n =10–12 mice per group (9-week-old mice); male, n =6 mice per group (14-week-old mice). ( d ) Food intake. n =5 male mice per group (10-week-old mice). ( e , f ) BAT and WAT mass. Female, n =10–12 mice per group (9-week-old mice); male, n =6 mice per group (14-week-old mice). P values (TG versus WT, two-tailed Student’s t -test) are indicated on top of the panels. ( g ) Liver, skeletal muscle and heart weights from mice in d . Gastro, gastrocnemius muscle; quad, quadriceps muscle. ( h ) Circulating triglycerides, free fatty acids and glucose levels. n =6–8 mice per group (14-week-old male mice). ( i ) miR-378 expression and BAT expansion in a second miR-378 transgenic line. n =6 mice per group (9-week-old male mice). * P <0.05, ** P <0.005 (two-tailed Student’s t -test). All data are mean±s.e. Full size image We performed Ki67 immunohistochemical staining on section of BAT at E16.5 or postnatal day 21. In either case, we found no apparent difference in preadipocyte proliferation between transgenic and control mice ( Supplementary Fig. 2A and B ). Overexpression of miR-378 in immortalized brown preadipocytes also had no effect on proliferation ( Supplementary Fig. 2C ). Our data suggest that BAT expansion is not due to an increase in preadipocyte proliferation. Instead, we hypothesized that miR-378 transgene promotes more preadipocytes to differentiate into adipocytes, and the preadipocyte pool is then rapidly replenished and maintained. miR-378 transgene enhances brown adipogenesis in vivo An increase of BAT mass can be attributed to cell number, cell size or both. Inspection of hematoxylin and eosin-stained BAT images ( Fig. 3a ) and estimation of nuclei densities (number of nuclei per unit area) ( Fig. 3b ) from these images suggested similar cell size between the transgenic and control mice, though the transgenic mice appeared to contain a slightly higher amount of lipid in BAT ( Fig. 3a ). Measurements of genomic DNA content revealed that BAT depots from the transgenic mice had a significantly higher cellularity ( Fig. 3c ). In contrast, the WAT adipocyte size in the transgenic mice was clearly smaller ( Fig. 3a ), and genomic DNA content per depot was similar compared with control mice ( Fig. 3c ). These results suggest that the expansion of BAT mass in the miR-378 transgenic mice is likely due to cell number, not cell size, whereas diminished WAT mass is likely due to cell size. Thus, ectopic expression of miR-378 in adipose promotes the formation of brown adipocytes but not white adipocytes, despite that both fat types express the miR-378 transgene. Furthermore, the shrinkage of white adipocyte might be secondary, caused by BAT expansion, which shifts the energy balance from storage to burning. Of note, the gradual increase of miR-378 level during adipogenesis ( Fig. 1d ) is consistent with its function, as similar expression profile has been observed for key adipogenic regulators such as Ppar γ. 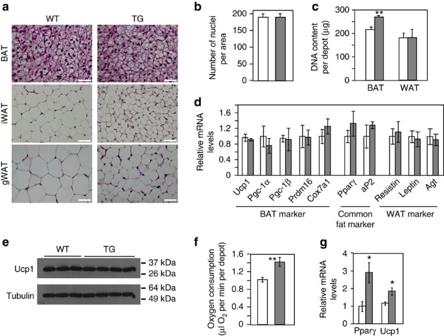Figure 3: miR-378 promotes brown adipogenesis but not white adipogenesisin vivo. (a) Hematoxylin and eosin staining for adipose tissue from 9-week-old male WT and TG mice. Scale bar, 50 μm. (b) Number of nuclei per BAT image. Twenty random images from three mice per group were counted, mean±s.e. (c) Genomic DNA content per fat depot;n=6 mice per group (11-week-old female mice), mean±s.e., **P=0.01 (two-tailed Student’st-test). (d) Expression of fat markers determined by real-time RT–qPCR in BAT;n=4–6 mice per group (9-week-old male mice), mean±s.e. (e) Immunoblotting showing Ucp1 protein levels in BAT (5-month-old female mice). (f) Measurement of oxygen consumption per BAT depot with a Clark-type oxygen electrode;n=4 mice per group (9-week-old female mice), mean±s.e., **P=0.01 (two-tailed Student’st-test). (g) Gene expression in BAT of neonatal mice determined by real-time RT–qPCR;n=3–6 mice per group, mean±s.e., *P<0.05 (two-tailed Student’st-test). Figure 3: miR-378 promotes brown adipogenesis but not white adipogenesis in vivo . ( a ) Hematoxylin and eosin staining for adipose tissue from 9-week-old male WT and TG mice. Scale bar, 50 μm. ( b ) Number of nuclei per BAT image. Twenty random images from three mice per group were counted, mean±s.e. ( c ) Genomic DNA content per fat depot; n =6 mice per group (11-week-old female mice), mean±s.e., ** P =0.01 (two-tailed Student’s t -test). ( d ) Expression of fat markers determined by real-time RT–qPCR in BAT; n =4–6 mice per group (9-week-old male mice), mean±s.e. ( e ) Immunoblotting showing Ucp1 protein levels in BAT (5-month-old female mice). ( f ) Measurement of oxygen consumption per BAT depot with a Clark-type oxygen electrode; n =4 mice per group (9-week-old female mice), mean±s.e., ** P =0.01 (two-tailed Student’s t -test). ( g ) Gene expression in BAT of neonatal mice determined by real-time RT–qPCR; n =3–6 mice per group, mean±s.e., * P <0.05 (two-tailed Student’s t -test). Full size image To ascertain that the expanded BAT is ‘true’ brown fat, not white fat-like, we analysed the expression of a number of fat markers in adult mice by RT–qPCR, which in principle measures relative expression level per cell. The mRNA levels of BAT-specific markers, common fat markers and WAT-specific marker were comparable between transgenic and control mice ( Fig. 3d ). As expected, Ucp1 protein levels remained unchanged as well ( Fig. 3e ). Moreover, the expanded BAT is fully functional, as indicated by ex vivo oxygen consumption assays ( Fig. 3f ). Our observation of no changes of common fat gene expression or BAT-specific gene expression is not unexpected; similar scenarios have been seen in BMP receptor ( Bmpr1a ) knockout [46] and aP2-Prdm16 transgenic mice [47] , respectively. It is possible that the normal differentiation process in vivo has already allowed a great extent of their expression that cannot be pushed further by the miR-378 transgene. Since brown adipocytes in neonatal mice are not as fully differentiated as those of adult mice, we wondered whether an effect of miR-378 on adipogenic gene expression would be observed at this early stage. Indeed, neonatal miR-378 transgenic mice displayed a higher expression of Ppar γ and Ucp1 ( Fig. 3g ). Taken together, our data strongly suggest that the expanded BAT is authentic and most likely retains its full range of molecular characteristics. BAT expansion suppresses formation of beige adipocytes iWAT expresses a considerable basal level of Ucp1 and displays high plasticity that is amendable to browning. We determined whether ectopic expression of miR-378 in this depot promotes the formation of beige adipocytes. In contrast to what we expect, basal levels of Ucp1 mRNA and protein, as well as expression of Prdm16 , which is a major regulator for BAT determination and beige adipocyte development [47] , [48] , were significantly decreased at room temperature ( Fig. 4a,b ), whereas levels of common adipogenic markers ( Ppar γ and aP2 ) remained normal. No change of Ucp1 in gonadal WAT was observed ( Supplementary Fig. 3A ). We envisioned that the expansion of BAT might cause a negative feedback response in iWAT. To investigate this further, we challenged the animals at 4 °C for 6 h. As expected, cold exposure induced Ucp1 expression in BAT of both wild-type and transgenic mice ( Supplementary Fig. 3B ) and in iWAT of wild-type mice ( Fig. 4a ). Strikingly, thermogenic pathway was completely blocked in iWAT of the transgenic mice, and Ucp1 expression was further suppressed at 4 °C ( Fig. 4a,c ). Consistent with this, we observed that Prdm16 level remained significantly lower and cold-induction of Pgc-1 α was severely impaired ( Fig. 4a,c ). We interpreted that high Ucp1 induction by cold in the expanded BAT somehow signals iWAT to curb its Ucp1 expression to maintain a normal and perhaps intrinsic cold response. Indeed, core body temperature was similar between the transgenic and control mice when shifted to 4 °C for 6 h ( Supplementary Fig. 3C ). 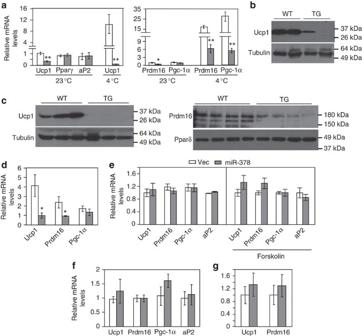Figure 4: BAT expansion, not miR-378per se, suppresses browning of subcutaneous iWAT. Empty bar, wild-type mice; grey bar, transgenic mice. (a)Ucp1,Prdm16andPgc-1α mRNA levels in iWAT from mice maintained at 23 °C or shifted to 4 °C for 6 h;n=4–6 mice per group (10-week-old male mice). WT versus TG: *P<0.05, **P<0.01 (two-tailed Student’st-test).Ucp1expression at 23 °C versus at 4 °C:P=0.009 for WT andP=0.001 for TG. Data are mean±s.e. (b) Immunoblotting of Ucp1 protein in iWAT from mice maintained at 23 °C (5-month-old female mice). (c) Immunoblotting of Ucp1 (left) and Prdm16 (right) protein in iWAT from 8-week-old male mice exposed to 4 °C for 6 h. (d)Ucp1,Prdm16andPgc-1α mRNA levels in iWAT from 8-week-old male mice treated with CL-316,243 for 5 days. Data were normalized to those of untreated wild-type mice;n=5–6 mice per group, mean±s.e., *P<0.05 (two-tailed Student’st-test). (e) iWAT preadipocytes from wild-type mice were infected with miR-378 or control lentiviruses and then differentiated. At day 6, adipocytes were either untreated or treated with forskolin (10 μM) for 5 h before harvesting (n=3, mean±s.e.). All data were relative to their respective controls. We typically observed that Ucp1 was induced to ~20-fold by forskolin relative to untreated adipocytes. (f) iWAT preadipocytes from wild-type mice and transgenic mice were differentiated. At day 6, adipocytes were harvested;n=4–6 mice per group, mean±s.e. (g) Real-time quantification ofUcp1andPrdm16mRNA levels in iWAT after interscapular BAT was removed;n=4 mice per group (9-week-old female mice), mean±s.e. Figure 4: BAT expansion, not miR-378 per se , suppresses browning of subcutaneous iWAT. Empty bar, wild-type mice; grey bar, transgenic mice. ( a ) Ucp1 , Prdm16 and Pgc-1 α mRNA levels in iWAT from mice maintained at 23 °C or shifted to 4 °C for 6 h; n =4–6 mice per group (10-week-old male mice). WT versus TG: * P <0.05, ** P <0.01 (two-tailed Student’s t -test). Ucp1 expression at 23 °C versus at 4 °C: P =0.009 for WT and P =0.001 for TG. Data are mean±s.e. ( b ) Immunoblotting of Ucp1 protein in iWAT from mice maintained at 23 °C (5-month-old female mice). ( c ) Immunoblotting of Ucp1 (left) and Prdm16 (right) protein in iWAT from 8-week-old male mice exposed to 4 °C for 6 h. ( d ) Ucp1 , Prdm16 and Pgc-1 α mRNA levels in iWAT from 8-week-old male mice treated with CL-316,243 for 5 days. Data were normalized to those of untreated wild-type mice; n =5–6 mice per group, mean±s.e., * P <0.05 (two-tailed Student’s t -test). ( e ) iWAT preadipocytes from wild-type mice were infected with miR-378 or control lentiviruses and then differentiated. At day 6, adipocytes were either untreated or treated with forskolin (10 μM) for 5 h before harvesting ( n =3, mean±s.e.). All data were relative to their respective controls. We typically observed that Ucp1 was induced to ~20-fold by forskolin relative to untreated adipocytes. ( f ) iWAT preadipocytes from wild-type mice and transgenic mice were differentiated. At day 6, adipocytes were harvested; n =4–6 mice per group, mean±s.e. ( g ) Real-time quantification of Ucp1 and Prdm16 mRNA levels in iWAT after interscapular BAT was removed; n =4 mice per group (9-week-old female mice), mean±s.e. Full size image This negative response could be due to either suppression of sympathetic tone into iWAT or due to suppression of β3-adrenergic signal transduction within iWAT adipocytes. To distinguish these possibilities, we intraperitoneally injected agonist CL-316243 daily for 5 days into miR-378 transgenic and littermate control mice. While levels of Ucp1 and Prdm16 were induced to fourfold and twofold, respectively, in the iWAT of control mice compared with untreated control mice, β3-adrenergic agonist treatment failed to rescue their expression in the transgenic mice ( Fig. 4d ). These results suggest that the recipient site responsive to BAT expansion is likely to be located within the iWAT adipocytes. To rigorously test whether the above-observed phenotype was indeed through a crosstalk between BAT and iWAT and not caused by a cell autonomous effect of miR-378, we overexpressed miR-378 through lentiviral infection in primary iWAT preadipocytes isolated from wild-type C57BL/6 mice. Cells were differentiated into mature adipocytes under a standard differentiation protocol. Microscopic examination found no effect of miR-378 on adipogenesis (see below). We found that expression of Ucp1 , Prdm16 and Pgc-1 α was not affected by miR-378 expression ( Fig. 4e ). Similar data were obtained when cells were treated with forskolin ( Fig. 4e ); forskolin induced Ucp1 expression by ~20-fold relative to untreated adipocytes. In addition, we isolated iWAT preadipocytes from both miR-378 transgenic and control littermates and differentiated them into mature adipocytes. We found that Ucp1 , Prdm16 and Pgc-1 α were not downregulated in adipocytes of the transgenic mice ( Fig. 4f ). These results are in striking contrast to that observed in vivo , strongly supporting the idea that suppression of beige adipocyte development in vivo cannot be attributed to overexpression of miR-378 within iWAT. Finally, we surgically removed BAT from interscapular regions of transgenic and control mice, and then allowed the animals to recover for 10 days. We found that, after BAT removal, levels of Ucp1 and Prdm16 gene expression were no longer lower in the transgenic mice ( Fig. 4g ). Taken together, the data presented in Fig. 4 reveal a crosstalk between BAT and iWAT, in which BAT expansion robustly suppresses Ucp1 expression and formation of beige adipocytes in iWAT. This negative response is at least in part mediated by downregulation of Prdm16 . BAT expansion prevents both genetic and diet-induced obesity One important question is whether the expanded BAT is sufficient to prevent obesity, particularly in the face of a decreased basal Ucp1 expression in the iWAT. We first addressed this question using ob/ob mice, since these mice have low energy expenditure and their BAT depots become impaired with time. We crossed the miR-378 transgenic mice with the ob/ob mice. As shown in Fig. 5a , the miR-378 transgene completely reversed the obese phenotype. In fact, the body weights of the ob/ob mice with the miR-378 transgene were similar to those of age-matched wild-type mice. The miR-378 transgene also improved BAT morphology and rescued hepatic steatosis in the ob/ob mice ( Fig. 5b ). Next, we fed the miR-378 transgenic mice and wild-type littermates with a high-fat diet. Their body weights, which were similar before high-fat diet, started to be significantly segregated at week 3 of high-fat diet feeding ( Fig. 5c ). At week 13, the control mice gained 22.4±0.9 g of body weight, while the transgenic mice only gained 10.3±0.8 g, which is equivalent to a typical body weight gain under a chow diet, although similar amounts of food were consumed ( Fig. 5d ). The body weight difference was due to massive reduction of WAT mass in the transgenic mice ( Fig. 5e ) that are associated with amelioration of adipocyte hypertrophy ( Supplementary Fig. 4 ). Taken together, we conclude that BAT expansion in the transgenic mice not only overcomes the negative response in iWAT, but also expends far more energy, leading to a complete prevention of both genetic and high-fat diet-induced obesity. 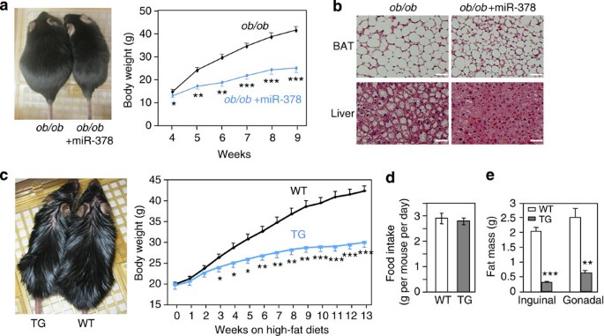Figure 5: miR-378-directed BAT expansion is sufficient to protect against both genetic and high-fat diet-induced obesity. (a) Left, representatives ofob/obmice andob/obmice carrying the miR-378 transgene at 9 weeks of age; Right, body weights ofob/obmice (n=7 mice) andob/obmice with the miR-378 transgene (n=4 mice) fed a normal chow diet. Mean±s.e., *P<0.05, **P<10−4, ***P<10−5(two-tailed Student’st-test). (b) Amelioration of liver steatosis and reduction of BAT lipid accumulation by miR-378 inob/obmice. Scale bar, 50 μm. (c) Six-week-old male mice were fed a high-fat diet for 13 weeks. Left, representatives of wild-type (WT) and transgenic (TG) mice after a 13-week high-fat diet; Right, body weights were measured weekly;n=8–9 mice per group, mean±s.e., *P<10−3, **P<10−4, ***P<10−6(two-tailed Student’st-test). (d) Consumption of high-fat diet by wild-type (WT) and transgenic (TG) mice;n=5 mice per group (10-week-old male mice), mean±s.e. (e) Inguinal and gonadal WAT mass of mice inc. Mean±s.e., **P<10−4, ***P<10−6(two-tailed Student’st-test). Figure 5: miR-378-directed BAT expansion is sufficient to protect against both genetic and high-fat diet-induced obesity. ( a ) Left, representatives of ob/ob mice and ob/ob mice carrying the miR-378 transgene at 9 weeks of age; Right, body weights of ob/ob mice ( n =7 mice) and ob/ob mice with the miR-378 transgene ( n =4 mice) fed a normal chow diet. Mean±s.e., * P <0.05, ** P <10 −4 , *** P <10 −5 (two-tailed Student’s t -test). ( b ) Amelioration of liver steatosis and reduction of BAT lipid accumulation by miR-378 in ob/ob mice. Scale bar, 50 μm. ( c ) Six-week-old male mice were fed a high-fat diet for 13 weeks. Left, representatives of wild-type (WT) and transgenic (TG) mice after a 13-week high-fat diet; Right, body weights were measured weekly; n =8–9 mice per group, mean±s.e., * P <10 −3 , ** P <10 −4 , *** P <10 −6 (two-tailed Student’s t -test). ( d ) Consumption of high-fat diet by wild-type (WT) and transgenic (TG) mice; n =5 mice per group (10-week-old male mice), mean±s.e. ( e ) Inguinal and gonadal WAT mass of mice in c . Mean±s.e., ** P <10 −4 , *** P <10 −6 (two-tailed Student’s t -test). Full size image We performed indirect calorimetry measurements in adult mice that were fed a normal chow diet or a 3-day high-fat diet, with conditions that transgenic and control mice had similar body weights. These studies confirmed our earlier results of no difference in food intake, and showed transgenic mice tended to be less active at night phase, although no statistical significance was reached ( Supplementary Fig. 5 ), suggesting that resistance to obesity is not due to potential decreased food intake or increased activity. Interestingly, we did not observe any difference in oxygen consumption or respiratory exchange ratio ( Supplementary Fig. 5 ), despite that BAT depot ex vivo on a per mouse basis had a higher oxygen consumption ( Fig. 3f ). Other mouse models that display changes in oxidative metabolism in adipose tissue or skeletal muscle but no difference in oxygen consumption and/or respiratory exchange ratio have been reported [49] , [50] , [51] . It has been discussed that a small difference in energy expenditure that is beyond the detection limit of indirect calorimetry could result in body weight difference over a long term [52] . miR-378 targets Pde1b in BAT but not in WAT We sought to understand the molecular mechanism by which miR-378 promotes BAT expansion. Targetscan ( www.targetscan.org ) predicts Pde1b , a Pde that catalyses the turnover of cAMP and cGMP [25] , to be a potential miR-378 target. cAMP and cGMP are signalling molecules that potentiate adipocyte differentiation [21] , [22] , [23] , [53] . Pde1b appeared to be ubiquitously expressed with a higher level in WAT than in BAT ( Supplementary Fig. 6A ). Pde1b level was initially decreased and then increased during brown adipogenesis ( Supplementary Fig. 6B ). Interestingly, single-nucleotide polymorphisms in the Pde1b gene were found to be associated with cattle backfat thickness [54] , [55] . The target sequence at the 3′ UTR of Pde1b is well conserved in mammals ( Fig. 6a ). We found that both endogenous Pde1b mRNA and protein in the BAT of transgenic mice were significantly decreased ( Fig. 6b,c ). To test whether Pde1b is a direct target of miR-378, we generated a luciferase reporter containing, at its downstream, either a wild-type 3′ UTR of mouse Pde1b or a variant in which the target sequence was mutated. We transfected these reporters into HEK293 cells. We found that the mutant reporter had a significantly higher activity than the wild-type reporter ( Fig. 6d ), most likely due to the presence of endogenous miR-378, which has a well-conserved sequence in human genome. Indeed, transfection of HEK293 cells with the miR-378 inhibitor increased the activity of the wild-type reporter but had no effect on the mutant reporter ( Fig. 6d ). These results demonstrated that Pde1b is a direct target of miR-378 in BAT. 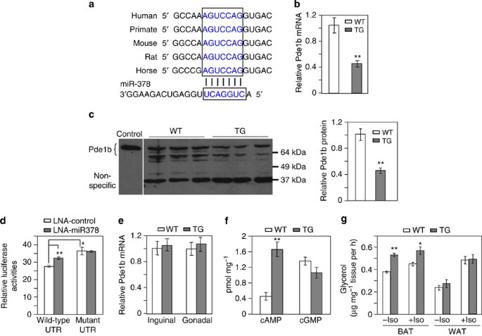Figure 6: BAT-specific suppression ofPde1bby miR-378. (a) Conserved miR-378 targeting sequence atPde1b3’ UTR. (b)Pde1bmRNA is downregulated in BAT of miR-378 transgenic mice;n=5 mice per group (9-week-old male mice), mean±s.e., **P<0.001 (two-tailed Student’st-test). (c) Pde1b protein levels in BAT from 5-week-old female WT and TG mice. Cell extracts from HEK293 cells transfected with a full-lengthPde1b1plasmid were used as a control to indicate the position of endogenous mousePde1b. BAT produces two expected major splice variants of Pde1b (Pde1b1 and Pde1b2) differing in their amino-termini70. Right panel shows quantification of the western blot. Mean±s.e., **P=0.005 (two-tailed Student’st-test). (d) HEK293 cells were transfected with locked nucleic acid (LNA) miR-378 inhibitor and a luciferase reporter carrying 3′ UTR ofPde1bas described in the online Methods. Luciferase activity was measured;n=3, mean±s.e., *P<0.05, **P<0.001 (two-tailed Student’st-test). (e) RelativePde1bmRNA level in inguinal and gonadal WAT of the transgenic mice;n=5 mice per group (9-week-old male mice), mean±s.e. (f) cAMP and cGMP levels in BAT;n=7 mice per group (9-week-old male mice), mean±s.e., **P<0.001 (two-tailed Student’st-test). (g) BAT and WAT lipolysis with or without 10 μM isoproterenol;n=5 mice per group (5-month-old male mice), mean±s.e., **P<0.0005, *P=0.012 (two-tailed Student’st-test). Figure 6: BAT-specific suppression of Pde1b by miR-378. ( a ) Conserved miR-378 targeting sequence at Pde1b 3’ UTR. ( b ) Pde1b mRNA is downregulated in BAT of miR-378 transgenic mice; n =5 mice per group (9-week-old male mice), mean±s.e., ** P <0.001 (two-tailed Student’s t -test). ( c ) Pde1b protein levels in BAT from 5-week-old female WT and TG mice. Cell extracts from HEK293 cells transfected with a full-length Pde1b1 plasmid were used as a control to indicate the position of endogenous mouse Pde1b . BAT produces two expected major splice variants of Pde1b (Pde1b1 and Pde1b2) differing in their amino-termini [70] . Right panel shows quantification of the western blot. Mean±s.e., ** P =0.005 (two-tailed Student’s t -test). ( d ) HEK293 cells were transfected with locked nucleic acid (LNA) miR-378 inhibitor and a luciferase reporter carrying 3′ UTR of Pde1b as described in the online Methods. Luciferase activity was measured; n =3, mean±s.e., * P <0.05, ** P <0.001 (two-tailed Student’s t -test). ( e ) Relative Pde1b mRNA level in inguinal and gonadal WAT of the transgenic mice; n =5 mice per group (9-week-old male mice), mean±s.e. ( f ) cAMP and cGMP levels in BAT; n =7 mice per group (9-week-old male mice), mean±s.e., ** P <0.001 (two-tailed Student’s t -test). ( g ) BAT and WAT lipolysis with or without 10 μM isoproterenol; n =5 mice per group (5-month-old male mice), mean±s.e., ** P <0.0005, * P =0.012 (two-tailed Student’s t -test). Full size image Interestingly, Pde1b mRNA expression remained unchanged in both inguinal and gonadal WAT of miR-378 transgenic mice ( Fig. 6e ). These results might, in part, explain the lack of WAT expansion, and suggest that targets of miR-378 are highly tissue- or cell type-specific. In support of this notion, we found that none of the other known miR-378/378* targets identified in other tissues, including Igf1r (cardiomyocytes) [56] , Crat and Med13 (liver) [57] , and ERR γ (cancer cells) [58] , was downregulated by the miR-378/378* transgene in BAT ( Supplementary Fig. 7 ), consistent with the idea that one microRNA can have distinct and tissue-specific functions through targeting different mRNAs [34] , [36] , [37] . We next determined whether reduction of Pde1b modulates cAMP and cGMP levels in BAT. We found that cAMP level was increased to more than 3.6-fold in the miR-378 transgenic mice, whereas cGMP level was not significantly different ( Fig. 6f ). Thus, Pde1b appears to predominantly regulate cAMP turnover in BAT, and cGMP level is refractory to changes of Pde1b . Our results suggest that suppression of Pde1b by miR-378 and hence elevation of cAMP level might be part of the mechanism underlying BAT expansion. An elevation of cAMP level is expected to lead to an increase of lipolysis in BAT. Since the process of isolation of single mature adipocytes might disturb intracellular cAMP content, we tested this idea in BAT tissue samples ex vivo . We found that lipolysis was indeed significantly higher in BAT of transgenic mice relative to control littermates ( Fig. 6g ). No difference was observed in WAT, consistent with the data that Pde1b was not downregulated in this adipose type. Interestingly, application of isoproterenol produced little and a slight increase of lipolysis in BAT of transgenic and control mice, respectively, but strongly enhanced lipolysis of WAT in both genotypes, which might be related to their respective preexisting basal β-adrenergic activation state. Increased lipolysis in BAT of transgenic mice did not cause an increase of plasma free fatty acids under both normal chow ( Fig. 2h ) and high-fat diet conditions ( Supplementary Fig. 8 ), indicating that released lipids are probably oxidized locally. miR-378 and Pde1b inversely regulates adipogenesis in vitro Given that miR-378 expression promotes BAT adipogenesis in vivo , we determined whether this effect can be recapitulated in vitro . We first performed our experiments in C3H10T1/2 mesenchymal stem cells. In a standard adipogenic assay condition that contains the general Pde inhibitor IBMX, we found that ectopic expression of miR-378/378* had little stimulatory effect on adipogenesis ( Supplementary Fig. 9A ). Removal of IBMX abrogated adipogenesis ( Supplementary Fig. 9B ). Importantly, expression of miR-378/378* strongly promoted the formation of adipocytes in the absence of IBMX, that is, a much higher percentage of cells were differentiated into adipocytes ( Fig. 7a,b ). Because of the increased number of adipocytes, levels of adipogenic markers, when assayed in the C3H10T1/2 population, were increased as well ( Fig. 7c ). Thus, miR-378 does positively regulate adipocyte differentiation in vitro , an effect that is masked by IBMX, further linking miR-378 to Pde1b . Accordingly, we infected C3H10T1/2 cells with Pde1b shRNA or scramble lentiviruses and differentiated them into adipocytes in the absence of IBMX. As shown in Fig. 7d,e , knockdown of Pde1b phenocopied miR-378 expression. 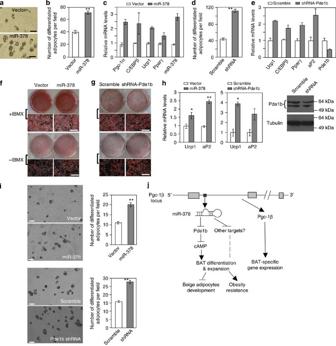Figure 7: miR-378 and Pde1b inversely regulate adipogenesisin vitro. (a–c) Ectopic expression of miR-378 promotes adipogenesis in C3H10T1/2 cells in the absence of Pde enzyme inhibitor IBMX. Experiments were repeated three times. Scale bar, 100 μm. Inb, number of differentiated adipocytes per field. Twenty fields were counted per condition. Mean±s.e., **P<10−5(two-tailed Student’st-test). Inc, real-time qPCR was used to detect gene expression of differentiation-dependent adipogenic markers. (d,e) Knockdown ofPde1bphenocopies the effect of miR-378 overexpression in the absence of IBMX. Ind, number of differentiated adipocytes per field. Twenty fields were counted per condition. Mean±s.e. **P<10−5(two-tailed Student’st-test). Ine, expression of differentiation-dependent adipogenic markers. (f) Adipogenesis of immortalized brown preadipocytes expressing miR-378. Experiments were repeated three times. Scale bar, 50 μm. (g) Adipogenesis of immortalized brown preadipocytes withPde1bknockdown. Experiments were repeated three times. In bothfandg, dark areas in microscopic images are undifferentiated preadipocytes. Scale bar, 50 μm. (h) RelativeUcp1andaP2mRNA levels in brown adipocytes generated as described infandg;n=3, mean±s.e., *P<0.05, **P<0.01 (two-tailed Student’st-test). Pde1b protein level was shown in brown adipocytes differentiated at a standard condition. (i) Ectopic expression of miR-378 or knockdown ofPde1bin primary brown preadipocytes increases the number of adipocytes during differentiation in the absence of IBMX. Scale bar, 50 μm. Mean±s.e., **P<10−6(two-tailed Student’st-test). (j) A model for miR-378 action in classical BAT. miR-378 controls brown adipogenesis and expansion in part through downregulatingPde1band hence elevating cAMP content, whereas the host genePgc-1β controls BAT-specific gene expression but not adipogenesisper se44. Figure 7: miR-378 and Pde1b inversely regulate adipogenesis in vitro . ( a – c ) Ectopic expression of miR-378 promotes adipogenesis in C3H10T1/2 cells in the absence of Pde enzyme inhibitor IBMX. Experiments were repeated three times. Scale bar, 100 μm. In b , number of differentiated adipocytes per field. Twenty fields were counted per condition. Mean±s.e., ** P <10 −5 (two-tailed Student’s t -test). In c , real-time qPCR was used to detect gene expression of differentiation-dependent adipogenic markers. ( d , e ) Knockdown of Pde1b phenocopies the effect of miR-378 overexpression in the absence of IBMX. In d , number of differentiated adipocytes per field. Twenty fields were counted per condition. Mean±s.e. ** P <10 −5 (two-tailed Student’s t -test). In e , expression of differentiation-dependent adipogenic markers. ( f ) Adipogenesis of immortalized brown preadipocytes expressing miR-378. Experiments were repeated three times. Scale bar, 50 μm. ( g ) Adipogenesis of immortalized brown preadipocytes with Pde1b knockdown. Experiments were repeated three times. In both f and g , dark areas in microscopic images are undifferentiated preadipocytes. Scale bar, 50 μm. ( h ) Relative Ucp1 and aP2 mRNA levels in brown adipocytes generated as described in f and g ; n =3, mean±s.e., * P <0.05, ** P <0.01 (two-tailed Student’s t -test). Pde1b protein level was shown in brown adipocytes differentiated at a standard condition. ( i ) Ectopic expression of miR-378 or knockdown of Pde1b in primary brown preadipocytes increases the number of adipocytes during differentiation in the absence of IBMX. Scale bar, 50 μm. Mean±s.e., ** P <10 −6 (two-tailed Student’s t -test). ( j ) A model for miR-378 action in classical BAT. miR-378 controls brown adipogenesis and expansion in part through downregulating Pde1b and hence elevating cAMP content, whereas the host gene Pgc-1 β controls BAT-specific gene expression but not adipogenesis per se [44] . Full size image We next tested our model in immortalized brown preadipocytes. Again, same number of preadipocytes were plated for control and experimental conditions, and were subjected to differentiation. In agreement with what was observed in C3H10T1/2 cells, neither miR-378 overexpression nor Pde1b knockdown had any effect in the presence of IBMX, while both of these two manipulations promoted formation of adipocytes in the absence of IBMX ( Fig. 7f,g ). Again, increased number of adipocytes was associated with higher adipogenic gene expression ( Fig. 7h ). In contrast, iWAT preadipocyte differentiation was not affected by miR-378 expression ( Supplementary Fig. 9C ). Finally, we performed adipogenesis experiments in primary brown adipocytes. We initially used brown preadipocytes from transgenic and control littermates. However, we found that individual animals displayed considerable variations in terms of both proliferation and differentiation capacities in vitro , even these brown preadipocytes were isolated from equal BAT mass and same genotype, thus precluding us to critically evaluate in vitro adipogenesis. To circumvent this problem, we isolated primary brown preadipocytes from wild-type C56BL6 mice, pooled them together and cultured them. Equal numbers of preadipocytes were infected with lentiviruses, selected with puromycin and amplified. Cells were then replated at equal numbers and differentiated without IBMX. Because of this relatively long procedure and lack of IBMX, cells lost their differentiation ability considerably, but we were able to reproducibly observe a significant increase of adipocyte number in these primary cells with either miR-378 ectopic expression or Pde1b knockdown ( Fig. 7i ). Together, our data show that miR-378 promotes brown adipocyte formation both in vivo and in vitro , and this is likely to be mediated, at least in part, through downregulation of Pde1b . Our studies have made the following discoveries: (1) miR-378 promotes brown adipogenesis, and as a result, transgenic expression of miR-378 in adipose tissue leads to the expansion of classical BAT but not of WAT; (2) BAT expansion is achieved at least, in part, through fat type-specific Pde1b downregulation and hence elevation of cAMP content; (3) BAT expansion suppresses development of beige adipocytes in iWAT; (4) BAT expansion alone is sufficient to prevent both genetic and high-fat diet-induced obesity, even in the face of decreased activity of beige adipocytes. Our work identifies miR-378 and Pde1b axis as a potential major molecular node that fine-tunes BAT mass and regulates systematic metabolism, and provides new insights into our understanding of BAT development and crosstalk between BAT and WAT. It is important to note that this miR-378 and Pde1b axis appears to be physiologically relevant, as BAT expansion and associated phenotypes requires a merely two- to threefold increase of miR-378 expression, and knockdown of Pde1b promotes adipocyte differentiation. The process of adipogenesis per se is largely shared by both brown and white adipocytes, and many adipogenic regulators and signalling pathways have been found to impact differentiation of both fat cell types. Nevertheless, studies in recent years have identified a number of genes that selectively promote brown adipogenesis [26] , [27] , [28] , [29] , [30] , [31] , [32] . We now extend this group of genes to include a microRNA. Previous investigations by others have demonstrated key roles of miRNAs in the inhibition of brown adipogenesis or enhancement of both brown and white adipogenesis [38] , [39] , [40] , [41] , [42] , [59] . To our knowledge, miR-378 is the first miRNA, shown to date, that selectively promotes brown adipogenesis. We reveal that miR-378 directly targets Pde1b in BAT, but not in WAT, to increase intracellular cAMP content, providing a plausible molecular mechanism for BAT expansion. It is noteworthy that the BAT expansion phenotype driven by miR-378 is reminiscent of that of the aP2-Foxc2 transgenic mice, which sensitizes cAMP signalling in adipose tissue [60] . Moreover, our proposed mechanism is strongly supported by our in vitro experiments showing that effects of miR-378 and Pde1b on brown adipogenesis are only manifested when Pde inhibitor IBMX is removed. Interestingly and similar to what we observed, miR-378 was previously not found to increase the number of adipocyte formation of ST2 mesenchymal precursor cells in the presence of IBMX; however, adipogenesis was not examined in the absence of IBMX in this early study [61] . While IBMX is widely used to inhibit Pde activity for efficient adipogenesis in vitro , the specific Pde enzyme involved in brown adipogenesis has not been firmly identified. Experiments performed a decade ago have led Nedergaard and co-workers to postulate that Pde1 might be important for inhibition of intracellular cAMP accumulation in brown adipocytes [62] . Their studies, together with our results presented here, suggest a potential critical negative role of Pde1b in the control of cAMP level and brown adipogenesis. Furthermore, our work elucidates an endogenous pathway attenuating Pde1b activity during brown adipogenesis. Our observation of fat type-specific targeting of Pde1b by miR-378 is consistent with the notion that miRNAs confer target and functional specificity in different cell types or tissues [34] , [36] , [37] . Indeed, miR-378/378* has been shown to have several different functions, including lipogenesis in ST2 cells [61] , fatty acid oxidation in liver [57] , and apoptosis and hypertrophy in cardiomyocytes [56] , [63] . Although how exactly Pde1b is a preferred target of miR-378 in BAT but not in WAT is currently unknown, this selective miR-378 and Pde1b interaction is presumably determined by the overall availability and complexity of other Pde1b -targeting miRNAs, other mRNA targets of miR-378, and competing endogenous RNAs, as alluded in other systems [64] . Interestingly, Pde1b protein is readily detectable by our western blot analysis and appears to be abundantly expressed in BAT. Thus, BAT-enriched miR-378 is employed to counterbalance abundantly expressed Pde1b , a mechanism likely to be important for maintaining the flexibility of BAT to expand. Of course, it is entirely possible that this process also involves other miR-378 targets that remain to be identified. Surprisingly, we find that BAT expansion, not miR-378 per se , elicits a robust negative feedback response in subcutaneous iWAT that suppresses formation of beige adipocytes. Crosstalk between BAT and WAT is an emerging, interesting topic with two previous documentations in the literature, showing that ectopic expression of Ucp1 in WAT inhibits endogenous Ucp1 expression in BAT [65] , and that BAT paucity causes a compensatory induction of beige adipocytes in iWAT [46] . These studies together with ours suggest that functions of BAT and beige adipocytes are highly coordinated, and that brown–white fat communication is a two-way process and is capable of generating diverse responses. Moreover, depending on the nature of the response, distinct mechanisms can be utilized. For example, the induction of beige adipocytes is mediated by an increase of sympathetic input to iWAT [46] , whereas the suppression of beige adipocytes observed in our study appears to directly stem from iWAT adipocytes and Prdm16 reduction without the need to attenuate sympathetic input. Interestingly, recent work shows that WAT can cell-autonomously sense temperature to induce thermogenic gene program [66] . Currently, we do not know yet what signal is emanated from BAT and what molecular pathway in iWAT is responding, but our miR-378 animal model might be a useful tool to dissect this process. We initially anticipated that the negative response in iWAT would neutralize the effect of BAT expansion on energy homeostasis. Instead, we find that the miR-378 transgenic mice are completely protected from both genetic and high-fat diet-induced obesity, to an extent that is similar to a body gain by wild-type mice on a normal chow diet, suggesting that energy expenditure due to BAT expansion far exceeds its negative impacts on iWAT. Notably, the net increase of BAT mass (~25 mg) in our transgenic mice only accounts for about 0.1% of total body weight, but can dramatically shift the energy balance, consistent with the idea that BAT possesses tremendous fuel combusting capacity [67] . It is important to note that our work in no way discounts the importance of beige adipocytes in energy homeostasis; in fact, their metabolic benefits have already been demonstrated [47] , [50] . Our data do suggest that expansion of classical BAT alone is sufficient to achieve obesity resistance, even in the face of compromised beige adipocytes. Given the presence of classical BAT in adult humans and the conservation of miR-378 in human genome, targeting the miR-378 and Pde1b axis to expand BAT might be a potential strategy for the treatment of obesity and metabolic diseases. Alternatively, unlocking the exact cellular and molecular mechanisms of the iWAT negative response may provide us information on how to use beige adipocytes for the treatment. miRNA screen BAT and gonadal WAT were isolated from wild-type male C57BL6 mice ( n =5, 10-week-old mice) and total RNA was extracted using TRIzol. miRNAs were reverse transcribed using QuantiMir kit (System Biosciences, Cat#RA420A-1). A total of 688 miRNAs were screened using qPCR-based miRNA profiling kit (System Biosciences, Cat#RA670A-1). Data of their expression levels normalized with levels of U6 snoRNA were listed in Supplementary Data 1 . miRNAs that displayed a high enrichment in BAT versus WAT were selected and their expression in other tissues was further examined. Animals A 600 bp genomic fragment containing the miR-378 locus was amplified from the first intron of Pgc-1β, sequenced and fused downstream with the 5.4 kb aP2 promoter. The transgenic DNA fragment was gel-purified and injected into fertilized embryos harvested from C57BL/6 × SJL hybrid mice. Two independent transgenic lines, which show similar phenotypes, were obtained and backcrossed with C57BL/6 for at least three generations. Heterozygous leptin-deficient mice were purchased from Jackson Laboratory (Stock # 000632) and crossed with miR-378 transgenic mice to generate ob/ob mice and ob/ob mice carrying the miR-378 transgene. Normal diet containing 4% (w/w) fat and high-fat diet containing 35% (w/w) fat were purchased from Harlan Teklad and Bioserv (Product# F3282), respectively. Food consumption was measured daily for individually caged mice for 2 weeks. Circulating triglycerides and free fatty acids were measured with commercial kits (Sigma, Cat#TR0100). We placed mice in a 4 °C cold room for 6 h for cold challenging experiments. We intraperitoneally injected mice with β3 agonist CL-316243 (Tocris, Cat#1499) daily at 1 mg kg −1 body weight for 5 days. The Institutional Animal Care and Use Committee of the University of Massachusetts Medical School approved all the animal studies. Littermate controls were used in all the experiments. Cellularity To measure genomic DNA content, fat depots were excised, weighted and minced. Samples with equal amounts were digested with 10 mM Tris buffer (pH 7.5) containing protease K (0.4 mg ml −1 ), and genomic DNA was precipitated with ethanol. DNA content was calculated as per fat depot. Gene expression and western blot analyses Total RNA was extracted using TRIzol. Gene expression was measured by RT–qPCR, and normalized with internal controls. Primer sequences were listed in Supplementary Table 1 . For western blot analysis, adipose tissue samples with equal amounts were homogenized with a lysis buffer (100 mM NaCl, 50 mM Tris (pH 7.5), 0.5% Triton X-100, 5% (w/v) glycerol). Tissue lysates were quantified, separated by SDS–polyacrylamide gel electrophoresis, immunoblotted with antibodies to Ucp1 (Sigma #U6382, 1:2,000), tubulin (DSHB#E7-S, 1:10,000) and Pde1b (Abgent #AP11846B, 1:500). To measure levels of Prdm16 protein, iWAT tissue were obtained from 2-month old wild-type and transgenic mice that were exposed at 4 °C for 6 h. The tissues were chopped into small pieces and homogenized in cold cytoplasmic lysis buffer (10 mM HEPES pH 7.9,10 mM KCl, 0.1 mM EDTA, protease inhibitors and 1 mM phenylmethylsulphonyl fluoride) with dounce homogenization until a single-cell suspension was achieved. The cell suspensions were swollen for 15 min on ice and nuclei were released by vortex vigorously with supplementation of 0.625% NP-40 in lysis buffer. The nuclei were then recovered by centrifugation at 3,000 g for 5 min at 4 °C, subsequently resuspended in 150 μl buffer (20 mM HEPES pH 7.9, 0.4 M NaCl, 10% glycerol, 1 mM EDTA, protease inhibitors and 1 mM phenylmethylsulphonyl fluoride), and rocked at 4 °C for 30 min. The nuclear lysate was centrifuged at 16,000 g for 10 min at 4 °C and the supernatant was loaded to SDS–polyacrylamide gel electrophoresis after protein quantification. Prdm16 antibody was purchased from R&D Systems (AF6295, 1:500). Oxygen consumption assays Brown fat depots were weighed and chopped into small pieces. Portions with equal amount (30 mg) were suspended in 5 ml Dulbecco’s phosphate-buffered saline supplemented with 25 mM glucose, 1 mM pyruvate and 2% BSA, and respiration was measured with a biological oxygen monitor (YSI model 5300A). Oxygen consumption was calculated as per depot. Luciferase reporter assays Mouse Pde1b 3′ UTR (1.24 kb) was cloned from genomic DNA, and a variant was also generated in which point mutations at the miR-378 targeting sequences were introduced. Both fragments were verified by sequencing and were placed downstream of the luciferase gene in the pMIR-REPORT vector (Invitrogen). HEK293 cells in 48-well plates were first transfected with locked nucleic acid (LNA) miR-378 inhibitor (50 nM) or control oligos (50 nM; both from Exiqon), using lipofectamine 2000 (Invitrogen). The next day, cells were transfected with the luciferase reporters (50 ng) and CMV-β-galactosidase plasmids (150 ng). Luciferase activity was measured 48 h after the first transfection and normalized with β-galactosidase activity. cAMP and cGMP assays Commercial kits (KGE012 and KGE003, R&D Systems) were used and manufacturer’s instructions were followed. Briefly, BAT depot was weighed, and equivalent amount (~50 mg) was minced with scissors and then homogenized with a 1-ml-glass dounce tissue grinder in 500 μl 0.1 N HCl. Lysates were collected into Eppendorf tubes and centrifuged at 10,000 g for 10 min. Then 200 μl supernatant was transferred to new tubes, and mixed with 28 μl 1 N NaOH and 228 μl calibrator diluent RD5-55. Samples were centrifuged again at 10,000 g for 10 min, and 100 μl supernatant was used for assay. cAMP and cGMP levels were expressed as pmol mg −1 BAT. Lipolysis assays ex vivo BAT and iWAT depots were dissected from 4-month-old wild-type and transgenic mice. Small pieces of adipose tissue with similar weights (~50 mg) obtained from similar locations were incubated for 1 h at 37 °C without shaking in 500 μl of KRB buffer (12 mM HEPES pH 7.4, 121 mM NaCl, 4.9 mM KCl, 1.2 mM MgSO 4 and 0.33 mM CaCl 2 ) containing 2% FA free BSA and 0.1% glucose with or without 10 μM isoproterenol. Glycerol release was measured from incubation buffer using Free Glycerol Reagent (Sigma) and calculated as μg per mg tissue per hour. Adipogenesis in vitro C3H10T1/2 cells were obtained from ATCC. Immortalized brown preadipocytes were generated previously [68] . miR-378 overexpression and Pde1b knockdown plasmids along with control plasmids were packaged in lentiviral vector plenti-CMV/puro [69] and pSP108 (Addgene), respectively. Viruses were first titered in C3H10T1/2 cells and brown preadipocytes. Cells were then infected with equal number of viral particles, and selected with puromycin to generate pooled stable cells. Equal number of cells was replated at 70% confluency. The next day (day −2), cells were changed to medium containing 20 nM insulin and 1 nM 3,3′,5-triiodo- L -thyronine (differentiation medium). At day 0, differentiation was induced by culturing cells in differentiation medium supplemented with 0.5 μM dexamethasone and 0.125 mM indomethacin and with or without 0.5 mM IBMX as indicated for 48 h. After this induction period, cells were replenished with new differentiation medium every other day. Primary iWAT preadipocytes were isolated from 2-week-old C57BL6/J mice through collagenase digestion. iWAT adipogenesis was performed by culturing confluent cells in medium containing 850 nM insulin, 1 nM 3,3′,5-triiodo- L -thyronine, 0.5 μM dexamethasone, 0.125 mM indomethacin and with or without 0.5 mM IBMX. Differentiated iWAT adipocytes were either harvested for gene expression analysis or fixed for Oil Red O staining. Primary BAT preadipocytes were isolated from neonatal (day 1) wild-type C56BL6 mice through collagenase digestion. Cells were pooled together and plated. When cells reached 70% confluence, they were infected with lentiviruses and selected with 2 μg ml −1 puromycin. Cells were then trypsinized and equal number of cells was plated. Confluent cells were differentiated in a medium containing 850 nM insulin, 1 nM 3,3′,5-triiodo-L-thyronine, 0.5 μM dexamethasone and 0.125 mM indomethacin for 48 h, and then switched to a medium containing 20 nM insulin and 1 nM 3,3′,5-triiodo- L -thyronine for another 4 days. Oil red O staining Cells were fixed with 3.7% (W/V) formaldehyde for 15 min at room temperature and then stained with 0.3% (W/V) Oil Red O solution in 60% isopropyl alcohol for 1 h. The excess staining was removed by washing with water. Brown fat removal Surgery was performed in 2-month old wild-type and transgenic mice. Mice were anaesthetized with isofluorane via a vaporizer. The fur in the interscapular area was clipped and incisions were made around the brown fat depot and brown fat was removed. Wound clips were used to close the skin incision. Animals were allowed to recover for 10 days before RNA isolation. Statistical analysis Two-tailed Student’s t -test was used for statistical analysis. P <0.05 was considered significant. Data are presented as mean±s.e.m. Sample size was determined based on power analysis and standard practice. No data were excluded. Randomization and blinding strategy was used whenever possible. How to cite this article: Pan, D. et al . MicroRNA-378 controls classical brown fat expansion to counteract obesity. Nat. Commun. 5:4725 doi: 10.1038/ncomms5725 (2014).